Superlattice-based thin-film thermoelectric modules with high cooling fluxes In present-day high-performance electronic components, the generated heat loads result in unacceptably high junction temperatures and reduced component lifetimes. Thermoelectric modules can, in principle, enhance heat removal and reduce the temperatures of such electronic devices. However, state-of-the-art bulk thermoelectric modules have a maximum cooling flux q max of only about 10 W cm −2 , while state-of-the art commercial thin-film modules have a q max <100 W cm −2 . Such flux values are insufficient for thermal management of modern high-power devices. Here we show that cooling fluxes of 258 W cm −2 can be achieved in thin-film Bi 2 Te 3 -based superlattice thermoelectric modules. These devices utilize a p-type Sb 2 Te 3 /Bi 2 Te 3 superlattice and n-type δ-doped Bi 2 Te 3− x Se x , both of which are grown heteroepitaxially using metalorganic chemical vapour deposition. We anticipate that the demonstration of these high-cooling-flux modules will have far-reaching impacts in diverse applications, such as advanced computer processors, radio-frequency power devices, quantum cascade lasers and DNA micro-arrays. Thermoelectric modules have long been considered for cooling high-power electronic [1] , [2] , [3] , [4] , [5] and opto-electronic devices [6] , and there have been consistent efforts to improve the cooling flux values of thermoelectric modules in the past decade [7] , [8] , [9] , [10] , [11] , [12] , [13] , [14] , [15] . The maximum cooling flux q max of a thermoelectric module is defined as the maximum cooling flux that the thermoelectric module is capable of providing at a temperature difference across the module (Δ T ) of zero and is given by equation (1) [16] , [17] below. where S p and S n are the Seebeck coefficients of the p- and n-type elements, respectively, ρ p and ρ n are the electrical resistivities of the p- and n-type elements, respectively, T C is the temperature of the cold side of the thermoelectric module, f is the packing fraction and l is the thickness of the thermoelectric elements. Equation (1) shows that q max of the thermoelectric module depends on the thermoelectric material properties, the element thickness and the packing fraction. One approach for increasing q max is to develop thermoelectric materials with a high thermoelectric figure of merit ZT (refs 1 , 7 , 8 , 9 , 10 , 11 , 12 , 13 , 14 , 15 , 18 , 19 , 20 , 21 , 22 , 23 , 24 ), as defined in equation (2). where S , ρ , k and T are the Seebeck coefficient, electrical resistivity, thermal conductivity and absolute temperature, respectively. Significant progress has been made in recent years to increase ZT using nanostructured materials such as thin-film superlattices [1] , [18] , [25] , [26] , thick films of quantum-dot superlattices [14] and nanocomposites [7] , [8] , [9] . Alternatively, q max of the thermoelectric module can be increased by reducing the element thickness, as q max is inversely proportional to l (refs 1 , 18 , 26 ). However, the reduction of element thickness is limited by two factors: the synthesis method for the thermoelectric elements; and the electrical contact resistance between the thermoelectric elements and the copper trace. Electrical constant resistance has a marked impact on the performance of thin thermoelectric modules since the magnitude of the contact resistance can be comparable to that of thermoelectric element itself. Bulk thermoelectric materials cannot be thinned below a few hundred microns, resulting in the modest maximum cooling flux of approximately 10 W cm −2 (refs 27 , 28 ). Epitaxial semiconductor films can be grown much thinner, resulting in a higher maximum cooling flux for thin-film modules. As a point of reference, commercially available thin-film thermoelectric modules have elements that are approximately 20-μm thick and have maximum cooling fluxes around 100 W cm −2 (ref. 29 ). However, even the cooling flux of state-of-the art thermoelectric modules is insufficient for advanced thermal management application. For instance, heat generation in a silicon microprocessor is non-uniform, with localized heat flux possibly larger than 200 W cm −2 , and GaN-based transistors can produce hotspots with heat fluxes in excess of 1 kW cm −2 (refs 4 , 30 , 31 ). In this paper, we present thermoelectric module capable of producing a cooling flux of 258 W cm −2 , more than double that of the current state-of-the-art value. The enhancement in the module-level cooling flux is a result of thin (8.1 μm) Bi 2 Te 3 -based thin-film superlattice materials with high intrinsic ZT, the δ-doped n-type structure, and reduced electrical contact resistances (2.68 × 10 −7 Ω cm 2 for n-type and 1.36 × 10 −6 Ω cm 2 for p-type). 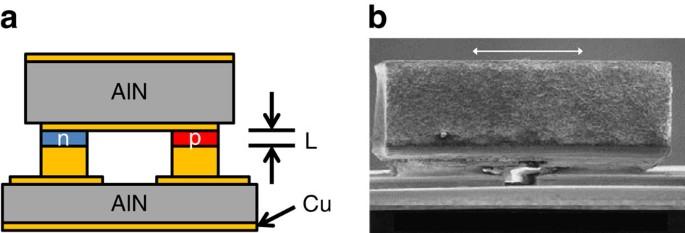Figure 1: Cross-sectional views of a Bi2Te3-based thin-film thermoelectric module. (a) Illustration of thin-film-based thermoelectric module, showing top and bottom AlN headers, Cu traces and n-type and p-type active elements.Lrepresents the length of the active elements, which is 8 μm in the present work. Figure is not to scale. (b) Scanning electron microscope image of the upper portion of a completed thin-film superlattice thermoelectric module. Scale bar, 250 μm. Material synthesis and module fabrication Figure 1a,b show the structure of the thermoelectric module. The thermoelectric material at the heart of the module consists of p-type 10/50 Å Bi 2 Te 3 /Sb 2 Te 3 superlattice and n-type δ-doped Bi 2 Te 3− x Se x , both of which are grown heteroepitaxially using metalorganic chemical vapour deposition [18] . The n-type structure is grown by periodically interrupting the growth of Bi 2 Te 3− x Se x and dosing the flow with Te and Se species. This δ-doping process can result in an increase in carrier concentration without a reduction in electron mobility. In the present experiment, 8.1-μm-thick thin films are grown and fabricated into cooling devices. Figure 1: Cross-sectional views of a Bi 2 Te 3 -based thin-film thermoelectric module. ( a ) Illustration of thin-film-based thermoelectric module, showing top and bottom AlN headers, Cu traces and n-type and p-type active elements. L represents the length of the active elements, which is 8 μm in the present work. Figure is not to scale. ( b ) Scanning electron microscope image of the upper portion of a completed thin-film superlattice thermoelectric module. Scale bar, 250 μm. Full size image The ZT values of the Bi 2 Te 3 /Sb 2 Te 3 superlattice materials used in this study have been previously measured by two different methods. One is the direct measurement of ZT by Harman method, which reported ZT>2 in ref. 18 . The second method is the determination of individual thermoelectric properties, such as Seebeck coefficient, electrical resistivity and thermal conductivity, followed by calculation of ZT. The ZT values of representative p- and n-type materials used in the devices in the present study were estimated, using this indirect technique, to be 1.4 and 1.5, respectively. These data have been added in Table 1 . These values were determined through measurement of the in-plane electrical resistivity and Seebeck coefficient of representative material along with an estimation of thermal conductivity via an in-couple-property-validation model. Details of this model are given in ref. 32 . Both direct measurement and indirect measurement of ZT were conducted at T =300 K. These estimated ZT values by the indirect method are slightly less than the ZT data measured directly via the Harman method for similar materials in ref. 18 . Table 1 ZT data from representative p- and n-type thermoelectric materials. Full size table In the device fabrication process, the top epitaxial surfaces of the p- and n-type materials are first metalized and then bonded to a common metalized AlN die header. Following chemical removal of the substrate, electrical contacts are fabricated on the exposed surface (typically with two n- and two p-type circular contacts designated as the 2N–2P configuration). This die header subassembly is then inverted and bonded to a second AlN header that contains the electrical traces used to power the module. As shown in Fig. 1b , the basic completed module structure has a 600 × 600-μm 2 top header area and is 550 μm tall. Electrical contact resistance One significant barrier to reaching high cooling fluxes with thin-film thermoelectric modules is electrical contact resistance between the metal electrodes and the thermoelectric elements, especially for Bi 2 Te 3 -based materials with low intrinsic electrical resistivity (10 −3 Ω cm) [1] , [26] . In the present experiment, two metallization methods (plated Au and evaporated Cr/Ni/Au metallization) and two different superlattice structures (standard structures and δ-doped structures) are explored to improve the electrical contact resistance. Au diffusion into the Bi 2 Te 3 lattice may very well be happening in the thermoelectric devices with plated Au contacts. The detailed effects of this potential Au diffusion need further study in the future. Electrical contact resistivity has been measured using the transmission line measurement technique [33] , which measures the resistance across an annular gap as a function of gap width, fabricated on a broad area of metallization on the top surface of the thin-film superlattice material. The metalized contacts are formed on the thin-film superlattice surface as shown in Fig. 2 , through the use of photoresist masks (gold is the metal contact, white is the thin-film superlattice surface) to form a set of six gaps with different gap widths. A four-wire probe is used to apply a small current across each gap (with two of the probe wires) and measure the voltage drop across the thin-film superlattice gap (with the other two probe wires). The gap resistance R g (measured Δ V over current) is a function of the gap width, governed by the relationship shown in equation (3). 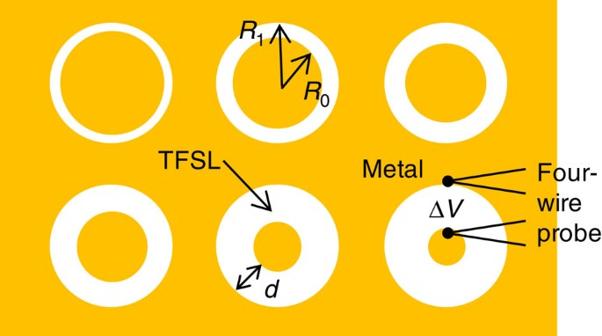Figure 2: Example of circular TLM patterns used for contact resistivity determination. In this measurement technique, six gaps of increasing widths (d=R1−R0) are patterned onto the sample surface. The gold colour represents the metal contact, while the white is the thin-film superlattice (TFSL) surface. A four-wire probe is used to apply a small current across each gap and measure the voltage drop (ΔV). Figure 2: Example of circular TLM patterns used for contact resistivity determination. In this measurement technique, six gaps of increasing widths ( d = R 1 − R 0 ) are patterned onto the sample surface. The gold colour represents the metal contact, while the white is the thin-film superlattice (TFSL) surface. A four-wire probe is used to apply a small current across each gap and measure the voltage drop (Δ V ). Full size image The gap resistance R g versus gap width d data is fitted to equation (3), with R s (sheet resistance) and L T (transfer length) as fitting parameters. Contact resistivity ρ c can then be calculated as R s × L T 2 with units of Ω m 2 . In the present modules, plated Au was used as the contact to the source (top) side of the n-type δ-doped Bi 2 Te 3− x Se x , while evaporated Cr/Ni/Au was used as the source (top) side of the p-type Sb 2 Te 3 /Bi 2 Te 3 . Plated Au was used as the sink (bottom) side contact of both the n- and p-type elements. Electric contact resistivity for thin-film superlattice materials and selected contact metals is shown in Table 2 . The R s , L T and ρ c values given in Table 2 are an average of the 6–8 experimental values measured for each material type and metallization scheme. The s.d. among these measurements is provided as well. Table 2 Specific electric contact resistivity, as measured by transmission line model (TLM) technique, for superlattice thermoelectric elements with different structures and metallization. Full size table Maximum temperature difference Δ T max To evaluate the maximum temperature difference Δ T max , the thermoelectric module is placed directly on a water-cooled heat sink, maintained at 25 °C, and the T C and T H values are measured using 25 μm diameter thermocouples as a function of current supplied to the module, I . The voltage V is also monitored as a function of electric current under vacuum (pressure, P <1 mTorr), up to the current producing the maximum Δ T max , which defines the current value of I max . The measured temperature difference and voltage behaviour of the thermoelectric module are given by [28] , [34] : In the above equations, S is the module Seebeck coefficient, which is determined by the voltage between the two electrical leads, V , and the temperature difference between the two AIN headers, Δ T . The module electric resistance is denoted by R , and consists of the electric resistance of the n and p elements R element , the electric resistance of the metal traces R trace , and the electric contact resistance between the elements and the metal traces R contact . The module electric resistance R can be determined by the voltage between the two electrical leads, V , and the electrical current I through the electrical leads. K is the module thermal conductance between the two AIN headers. R th is the parasitic thermal resistance of the module, which is the difference between the module thermal resistance and the thermal resistance of the n and p thermoelectric element pair ( Fig. 3 ). In the Δ T max measurements, there is no heat pumped by the module (cooling power, Q P =0) and the module parameter values can be determined by fitting equation (4) to the experimental Δ T as a function of I , V , T C and T H data, and similarly fitting equation (5) to the voltage data. The inclusion of a parasitic thermal resistance R th is necessary when considering thin-film thermoelectric modules, because the high-heat fluxes that occur within the module produce an internal element hot-side temperature T H int that is different from the externally measured value T H . 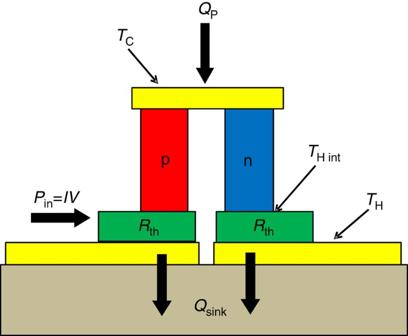Figure 3: Thin-film thermoelectric module structure. The red and blue rectangles represent the p- and n-type active TE materials, respectively. Yellow represents the current traces and tan represents the ceramic bottom header of the module. Heat entering the module is given byQP, while the heat being pumped out is given byQsink.TC,THandTH intare the cold-side temperature, externally measured hot-side temperature and internal element hot-side temperature, respectively. The green rectangles represent the parasitic thermal resistancesRth, which reduce the externally observed ΔTvalue. Figure is not drawn to scale. Figure 3: Thin-film thermoelectric module structure. The red and blue rectangles represent the p- and n-type active TE materials, respectively. Yellow represents the current traces and tan represents the ceramic bottom header of the module. Heat entering the module is given by Q P , while the heat being pumped out is given by Q sink . T C , T H and T H int are the cold-side temperature, externally measured hot-side temperature and internal element hot-side temperature, respectively. The green rectangles represent the parasitic thermal resistances R th , which reduce the externally observed Δ T value. Figure is not drawn to scale. Full size image The upper portion of Fig. 4 shows Δ T versus I data for the module with the largest contact diameter (230 μm). The circles indicate the experimental external Δ T values measured with thermocouples, and the curve drawn through these points is the fit of equation (4) to the data, using a parasitic thermal resistance of R th =(3.08±1.98) K W −1 . An external Δ T max value of 43.54 K is observed at an electric current of 14.8A, and the upper dashed curve shows the predicted internal Δ T ( T H int − T C ) occurring inside the module, which has a maximum value of 49.3, 5.7 K higher than the external value. The difference in internal and external Δ T is caused by the internal thermal resistance R th , which reduces the external Δ T that can be measured by the thermocouples. The multidimensional fit of equation (4) to experimental Δ T external versus I data also yields the values of the ratios S / K (0.0228 μV W −1 ) and R / K (0.349 Ω K W −1 ). 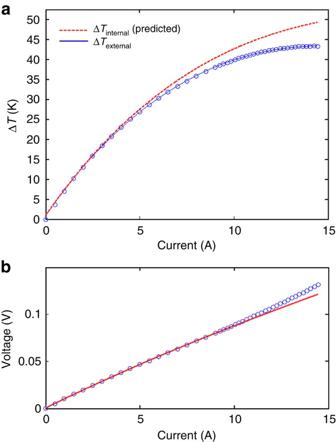Figure 4: Analysis of experimental data. (a) Experimental ΔTversusIdata for the module with the largest effective contact diameter (230 μm) and the fit of equation 4 to the data. Blue dots represent experimentally measured data points, and the blue line represents the fit . The red dotted line indicates predicted internal temperature difference (Thint−TC) versusI. (b) CorrespondingVversus I data for the same module. The blue dots represent experimentally measured data points, and the red line represents the theoretical fit. Figure 4: Analysis of experimental data. ( a ) Experimental Δ T versus I data for the module with the largest effective contact diameter (230 μm) and the fit of equation 4 to the data. Blue dots represent experimentally measured data points, and the blue line represents the fit . The red dotted line indicates predicted internal temperature difference ( T hint − T C ) versus I . ( b ) Corresponding V versus I data for the same module. The blue dots represent experimentally measured data points, and the red line represents the theoretical fit. Full size image Figure 4b shows the voltage versus current data for the same module. R can be determined via a one-dimensional least squares fit of equation (4) to this experimental V versus I data, which subsequently allows for the calculation of K and S from the previously determined R / K and S / K values. The resulting values of the total Seebeck coefficient S= (450±48) μV K −1 , thermal conductance K= (19.7±2.1) mW K −1 and electric resistance R= (6.87±0.01) mΩ are given in the legend of Fig. 4b . Details of this procedure have been described elsewhere [34] . Maximum cooling flux q max The cooling power for a thermoelectric module in the presence of a parasitic thermal resistance R th is shown in equation (6), where Δ T is the externally measured temperature difference [28] , [34] . In the case of R th =0, equation (6) reduces to the standard thermoelectric heat-pumping equation [35] , where the maximum cooling power Q P occurs when I=ST C /R (which is I max ). To determine I max in the case of non-zero R th , the voltage dependence in equation (6) is eliminated using equation (5), and after some rearrangement the expression for Q P becomes: Equation (7) is then differentiated with respect to I and solved numerically for the value of I that yields a zero of the resulting expression. The I max value is then substituted into equation (7), along with the individual fitted module parameter values to obtain the Q max value that is expected. The I max values calculated using equation (5) are found to agree with the experimentally observed values in these modules and are smaller than what is obtained from using the standard expression I max =ST C /R . The maximum cooling flux q max is calculated by dividing the total cooling power Q max by the top header area of the module, which is 600 × 600 μm 2 . The performance of four thin-film thermeoelctric modules with different contact diameters (that is, the packing fraction) is summarized in Table 3 . The table shows the measured maximum cooling flux ( q max =Q max /A T ), as well as the predicted value and a discrepancy of 13% is observed between the predicted and measured values. The coefficient of performance (COP) values were calculated at q max ; that is for Δ T= 0 K. With the establishment of the q max value and Δ T values, the load lines can be determined, as shown in Fig. 5 . Table 3 Performance of thin-film thermoelectric modules of varying contact diameter (that is, packing fraction). 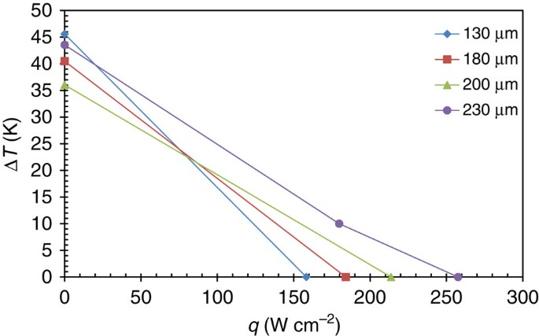Figure 5: Load lines for each of the four measured modules of this work. The load lines are determined by the measurement ofqmaxat ΔT=0K, and the measurement of ΔTmaxatq=0 W m−2. An additional data point for the case of ΔT=10 °C is included for the module with the largest contact diameter (230 μm). Full size table Figure 5: Load lines for each of the four measured modules of this work. The load lines are determined by the measurement of q max at Δ T =0K, and the measurement of Δ T max at q =0 W m −2 . An additional data point for the case of Δ T =10 °C is included for the module with the largest contact diameter (230 μm). Full size image In the case of the largest module, an additional data point that was obtained at Δ T= 10 °C is also shown. The maximum temperature difference Δ T max should not be dependent on the module geometry, but the variation seen indicates a possible undetermined parasitic phenomenon may be present. Further studies are needed to identify this undetermined parasitic phenomenon. It can be seen that a maximum cooling flux in excess of 250 W cm −2 is achieved in the thin-film Bi 2 Te 3 superlattice thermoelectric module with a contact diameter of 230 μm (that is, 48% packing fraction). This value is 25 times higher than is typically observed in commercial-off-the-shelf bulk thermoelectric modules ( http://www.marlow.com ) and more than 2.5 times better than commercial-off-the-shelf thin-film modules ( http://www.lairdtech.com ). The maximum cooling flux of the module was measured using two different methods, the Q-meter method by RTI and the non-contact IR method by University of Maryland. 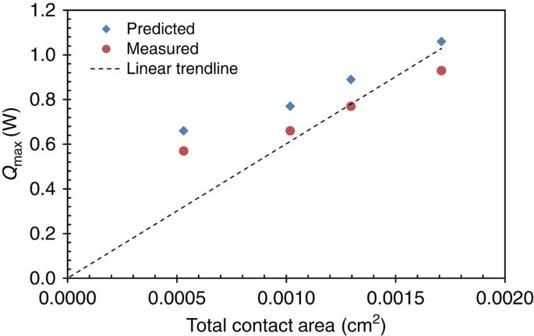Figure 6:Qmaxversus total contact area data for the four thin-film thermoelectric modules of this work. Experimentally measured values are represented by red squares, and the corresponding theoretically predicted values are represented by blue diamonds. The dotted line represents a linear trendline fit to the experimental data. This trendline has been indexed to the origin and is expressed by the equationy=601.6x. Contact diameter and packing fraction Figure 6 shows the dependence of maximum cooling power Q max as a function of the total element contact area A c (including both n and p contacts). The top header area A T is 600 × 600 μm 2 for all of the modules tested. The packing fraction is the ratio of the total element contact area A c to the top header area of the module A T , and the module with a contact diameter of 230 μm has a packing fraction of 48%. Figure 6: Q max versus total contact area data for the four thin-film thermoelectric modules of this work. Experimentally measured values are represented by red squares, and the corresponding theoretically predicted values are represented by blue diamonds. The dotted line represents a linear trendline fit to the experimental data. This trendline has been indexed to the origin and is expressed by the equation y =601.6 x . Full size image The calculated Q max values shown in Fig. 6 are consistently 12–14% larger than what is experimentally observed, which is likely due to other internal parasitic thermal resistances not accounted for in the model shown in equations (4) and (6). Specifically, the internal thermal resistance values that are used in these calculations are obtained using Δ T max measurements under the condition of no heat pumping ( Q P =0). In this case the only internal thermal resistance that the measurement is sensitive to is located below the thermoelectric elements, as indicated by R th in Fig. 3 . However, when heat is being pumped by the module through the top header, as is the case in these heat flux measurements ( Q P >0), any additional thermal resistances, such as thermal spreading resistance that occurs in the module regions above the thermoelectric elements will be important. This additional internal thermal resistance will further reduce the thermoelectric heat pumping in a manner similar to that seen for the lower internal thermal resistance. Capturing the additional internal thermal resistances in the model will reduce the calculated heat pumping and improve agreement between predicted and measured values. The basis for the larger cooling fluxes produced by thinner thermoelectric elements is the reduced electrical resistance of the thermoelectric structure, which in turn allows for the use of larger electrical currents. The higher currents produce more Seebeck heat pumping per unit area, as shown in equation (8). where Q P is the amount of heat pumped; S , R and K are the Seebeck coefficient, electrical resistance and thermal conductance of the thermoelectric module, respectively; T C and T H are the heat source and heat sink temperatures, respectively; I is electric current; n is the number of thermoelectric couples in the module; l is the thickness of one semiconductor leg; A is the cross-sectional area of one semiconductor leg (n and p are assumed to have identical geometry); and s , ρl/A and kA/l are the per-couple Seebeck coefficient, electrical resistance and thermal conductance, respectively. Equation (8) does not consider the parasitic thermal and electric resistance in the module. The input electrical current that corresponds to the case of max Q P can be calculated from the first derivative of the Q P =f ( I ) function and is equal to ST C /R . For bulk thermoelectric modules, the maximum value of Q P is low, because bulk thermoelectric material cannot be thinned below a thickness of few hundred microns, limiting the maximum current due to the high module electric resistance R . The electrical current limitation results in bulk thermoelectric heat-pumping capabilities in the 1–10 W cm −2 range. Epitaxial semiconductor films can be grown much thinner (for example, hundreds of nm), decreasing the electrical resistance and allowing larger electrical currents producing much higher cooling fluxes. For any given reduction in l by a factor of α , optimized I will increase by α . With all other things being equal, the cooling flux can be increased by a factor of 2, 5 or 10 times simply by decreasing the film thickness by a factor of 2, 5 or 10 times and increasing the electrical current accordingly. Theoretically, cooling fluxes, on the order of several hundred W cm −2 , can be achieved simply by thinning the thermoelectric material. However, there are several parasitic effects that need to be overcome to achieve the full potential of thin-film thermoelectric modules. The most significant barrier to high cooling fluxes is electrical contact resistance between metal electrodes and the semiconductor layers. In thin thermoelectric modules, the magnitude of the contact electric resistance can be comparable to the values of the resistance of the thermoelectric element itself, which will increase the total electric resistance of the module and reduce its maximum cooling flux. In this work, a low electric contact resistivity ρ c in the range of 1–2 × 10 −6 Ω cm 2 has been achieved, using the evaporation of Cr/Ni/Au to fabricate the metal electrodes as well as δ-doped superlattice structures. Further reduction to the order of 10 −8 Ω cm 2 is desired for thin-film thermoelectric module with element thickness <2 μm. Another barrier to wide adoption of thin-film thermoelectric modules is thermal resistances in the thermal management system. For heat flux values of several hundred W cm −2 , low thermal resistances, on the order of 0.03–0.05 cm 2 K W −1 , need to be present on both the hot and cold sides of the thermoelectric module for efficient integration of thermoelectric coolers into the system. In particular, a low thermal resistance present at the hot side takes the higher priority, due to the greater heat flow through the hot side, with Q hot = Q cold (1+1/COP). This requires more advanced heat exchangers and cold plates. Q-meter method for characterization of thin-film thermoelectric modules To evaluate the heat-pumping capacity, the thermoelectric modules are placed on top of a Q-meter ( Fig. 7 ), a metal post of known dimensions and thermal conductivity, used to determine the total heat flow passing through it by measuring the temperature gradient along its length. The Q-meter base is mounted to a water-cooled heat sink and the thermoelectric module is mounted to the top. The thermoelectric module is energized using a four-wire current–voltage measurement system employing thin Cu wires, approximately 2.5 cm long (either 250 or 500 μm in diameter), to connect the thermoelectric module to external instrumentation. Heat is applied to the top of the thermoelectric module using a resistive heater. The top and bottom thermoelectric module temperatures T C and T H , respectively, are read using 25 μm diameter thermocouples precisely positioned on the thermoelectric module. The entire system is operated under vacuum ( P <1 mTorr) to minimize convective losses. The water-cooled heat sink on the Q-meter is adjusted to maintain the thermoelectric hot-side temperature ( T H ) at about 25 °C. Since the test chamber is evacuated, convective losses are minimized. Thus, the heat flowing down the Q-meter is the sum of heat being pumped by the thermoelectric module, Q P , the electrical input power flowing into the thermoelectric module, P in and the thermal contribution of the four wires connecting the thermoelectric module to the external circuit, P wire ( Q meter = Q P + P in + P wire ). 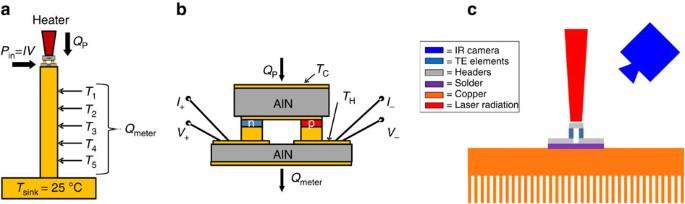Figure 7: Experimental arrangements for the measurement of heat pumped by the thermoelectric module. (a) Schematic of a thermoelectric module mounted on a Q-meter.T1throughT5represent the thermocouple measurements along the length of the Q-meter. (b) Schematic of a thermoelectric module showing the heat pumped by the module (QP) and additional contributions of the electrical input power (Pin) and wire conduction/heat generation (Pwire) to the heat measured by the Q-meter (Qmeter). The placement of the thermocouples on the cold side and hot side of the thermoelectric module is indicated byTCandTH, respectively. (c) Testing apparatus used to perform non-contact measurements of cooling fluxqand temperature difference ΔTof the thermoelectric modules. Figure 7: Experimental arrangements for the measurement of heat pumped by the thermoelectric module. ( a ) Schematic of a thermoelectric module mounted on a Q-meter. T 1 through T 5 represent the thermocouple measurements along the length of the Q-meter. ( b ) Schematic of a thermoelectric module showing the heat pumped by the module ( Q P ) and additional contributions of the electrical input power ( P in ) and wire conduction/heat generation ( P wire ) to the heat measured by the Q-meter ( Q meter ). The placement of the thermocouples on the cold side and hot side of the thermoelectric module is indicated by T C and T H , respectively. ( c ) Testing apparatus used to perform non-contact measurements of cooling flux q and temperature difference Δ T of the thermoelectric modules. Full size image Non-contact method for characterization of thin-film thermoelectric modules The performance of the thermoelectric modules was also characterized using the non-contact IR method. Figure 7c shows a schematic of the apparatus used for testing, consisting of a heat sink, the thermoelectric module, a laser and an infrared camera. The testing procedure consisted of first providing the thermoelectric module with electrical power, creating a temperature difference across the module. The laser was then used to heat the cold side of the thermoelectric module, decreasing the module-level Δ T . The laser power was gradually increased until the Δ T across the module was 0 K, indicating that the maximum heat pumping for that current had been reached. The process was repeated at several electrical powers to determine the electrical current that produced the maximum module heat pumping. The output power of the laser was determined using a calibration curve, which was created in situ , taking into account all loses in lenses and optical equipment. The emissivity of the cold side of the thermoelectric module was determined using the infrared camera, and from Kirchhoff’s law, the absorptivity of the cold side was assumed to be equal to the emissivity. Thus, the total amount of power being pumped through the module could be readily calculated. Nomenclature A Nomenclature table defining all of the variables used in this work is given in Supplementary Note 1 . How to cite this article: Bulman, G. et al . Superlattice-based thin-film thermoelectric modules with high cooling fluxes. Nat. Commun. 7:10302 doi: 10.1038/ncomms10302 (2016).